The pitfalls of interpreting hyperintense FLAIR signal as lymph outside the human brain 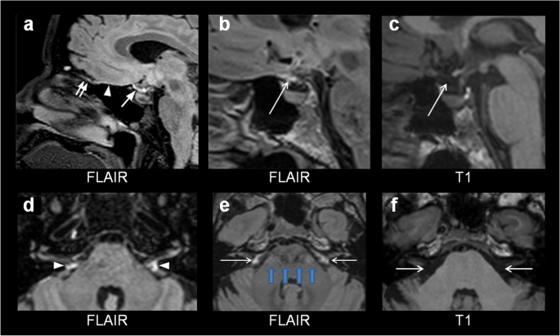Fig. 1: CSF flow artifacts at FLAIR in the subarachnoid space. aIn their Figure 4a, Albayram et al.3point at a linear hyperintensity at sagittal FLAIR in the suprasellar cistern and identify this as lymph.bImage from our same Prisma MRI scanner (Siemens, Erlangen) shows a similar phenomenon (arrow).cAt T1 weighted MRI through the same section it becomes clear that the FLAIR hyperintensity is within the CSF compartment (arrows), not the dura itself, which in this region is constituted by the sellar diaphragm immediately adjacent to the upper border of the pituitary gland. This clearly indicates a flow artifact derived from CSF pulsations within the suprasellar cistern.dIn their Figure 4f, Albayram et al.3point at FLAIR hyperintensities (arrowheads) within the cerebellopontine angle cisternal spaces and identify them as lymph (axial section).eWe reproduce similar findings (arrows) at our same MRI Prisma scanner (Siemens, Erlangen). Propagation of artifacts through the brain stem (blue arrows) in the same level (along the phase encoding direction), as also seen to a minor extent ind, is highly suggestive that these are CSF flow artifacts.fAt T1 weighted MRI through the same imaging plane it becomes clear that the hyperintensities at FLAIR correspond to the CSF space (arrows), not the dura or cranial nerves. The MRI shown in Fig. 1 was obtained as part of a study of patients undergoing diagnostic work-up of epilepsy, approved by The Regional Committee for Medical and Health Research Ethics (REK) of Health Region South-East, Norway (2020/121533), and was obtained after written and oral informed consent. We used a 3 Siemens Prisma MRI scanner with sequence parameters including the following: 1. 3D T1-gradient echo (T1-MPRAGE-ADNI): sagittal scanning plane; repetition time (TR) = 2300 ms; echo time (TE) = 2.93 ms; inversion time = 900 ms flip angle = 9°; 1 average; 1 mm isotropic voxels. 2. 3D T2-Fluid Attenuated Inversion Recovery (FLAIR): sagittal scanning plane; TR = 5000 ms; TE = 386 ms; inversion time = 1800 ms; flip angle = 120°; 1 average; 0.9 mm isotropic voxels Reporting summary Further information on research design is available in the Nature Portfolio Reporting Summary linked to this article.